Ultrafast optical demagnetization manipulates nanoscale spin structure in domain walls During ultrafast demagnetization of a magnetically ordered solid, angular momentum has to be transferred between the spins, electrons, and phonons in the system on femto- and picosecond timescales. Although the intrinsic spin-transfer mechanisms are intensely debated, additional extrinsic mechanisms arising due to nanoscale heterogeneity have only recently entered the discussion. Here we use femtosecond X-ray pulses from a free-electron laser to study thin film samples with magnetic domain patterns. We observe an infrared-pump-induced change of the spin structure within the domain walls on the sub-picosecond timescale. This domain-topography-dependent contribution connects the intrinsic demagnetization process in each domain with spin-transport processes across the domain walls, demonstrating the importance of spin-dependent electron transport between differently magnetized regions as an ultrafast demagnetization channel. This pathway exists independent from structural inhomogeneities such as chemical interfaces, and gives rise to an ultrafast spatially varying response to optical pump pulses. Demagnetization of a ferromagnet by an optical excitation pulse is known to proceed on an ultrafast timescale, typically in the femtosecond regime. Since the discovery of this ultrafast process by Beaurepaire et al . in 1996 (ref. 1 ), its mechanism has been intensely debated. So far, most work has focused on homogeneous samples to understand the intrinsic demagnetization mechanisms, with recent progress including the role of spin–orbit interaction and magnetocrystalline anisotropy [2] , [3] , the importance of electron–phonon-mediated spin-flip scattering [4] , and the interplay of different demagnetization time constants at different lattice sites in ferrimagnets [5] . A spatial component (beyond one unit cell), and hence possible additional extrinsic ultrafast demagnetization mechanisms, has entered the discussion so far only via ferromagnetic–paramagnetic (FM–PM) interfaces in thin-film samples [6] , [7] . Here, we report on experiments employing magnetic thin-film samples exhibiting a labyrinth-like network of oppositely-magnetized domains with structure sizes on the nanometre lengthscale. As this lengthscale is also relevant for the diffusion of photo-excited electrons [7] , changes in the domain spin structure during femtosecond demagnetization can be expected. To achieve the necessary temporal and spatial resolution, our pump-probe experiments were performed at the free-electron laser (FEL) FLASH [8] , [9] delivering intense, ~100 fs long soft X-ray pulses. Previous work combining high temporal and spatial sensitivity was either limited in spatial resolution due to the application of a far-field optical probe [5] , [10] , [11] or limited to the tens of picosecond time domain due to the picosecond X-ray pulses employed [12] . In the present study, we are able to detect magnetization changes on lengthscales of a few nanometres with a temporal resolution of 240 fs by analysing the changes in the magnetic scattering signal of the X-ray probe. As a result, the effects of spin diffusion become experimentally accessible in a spatio-temporally matched way. We show that spin diffusion opens a topography-dependent and hence extrinsic channel for ultrafast demagnetization as was predicted in simulations by Battiato et al . [7] . In contrast to the situation considered in refs 6 , 7 , in our experiments the demagnetization effect solely relies on the proximity of oppositely-magnetized domains without any necessity for chemical or structural inhomogeneity of the sample. Magnetic small-angle X-ray scattering We investigate the magnetic response to optical pumping for a lateral labyrinth-domain pattern in a thin-film Co/Pt multilayer sample as shown in Fig. 1a . Because of the strong magnetic interface anisotropy in this system, alternating 'up' and 'down' magnetic domains form in a self-organized manner, with magnetization parallel or antiparallel to the sample normal. Note that the sample is laterally homogeneous with respect to elemental composition, that is, the boundaries between differently magnetized regions are purely magnetic in nature and do not contain spacer layers disrupting the electronic band structure. 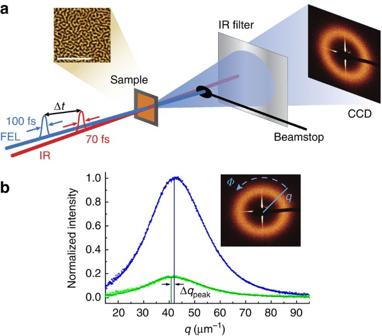Figure 1: Experimental set-up and data evaluation. (a) The magnetic multilayer sample is pumped by an optical laser pulse and probed by a delayed X-ray pulse produced by the FEL. The magnetic SAXS pattern is recorded on an IR-protected charge-coupled device (CCD) camera while the intense directly transmitted radiation is blocked by a beamstop. The inset shows a typical magnetic force micrograph of the sample in the probed labyrinth-domain state. The scale bar in the micrograph corresponds to 2 μm distance. (b) By fitting the azimuthally integrated (see inset) SAXS intensity, the intensity maximum is determined. We observe a decrease in the intensity and a shift of the peak position Δqpeak, when comparing unpumped (blue) and pumped (green) spectra (pump fluence: 14.2 mJ cm−2, time delay: 1.3 ps). Figure 1: Experimental set-up and data evaluation. ( a ) The magnetic multilayer sample is pumped by an optical laser pulse and probed by a delayed X-ray pulse produced by the FEL. The magnetic SAXS pattern is recorded on an IR-protected charge-coupled device (CCD) camera while the intense directly transmitted radiation is blocked by a beamstop. The inset shows a typical magnetic force micrograph of the sample in the probed labyrinth-domain state. The scale bar in the micrograph corresponds to 2 μm distance. ( b ) By fitting the azimuthally integrated (see inset) SAXS intensity, the intensity maximum is determined. We observe a decrease in the intensity and a shift of the peak position Δ q peak , when comparing unpumped (blue) and pumped (green) spectra (pump fluence: 14.2 mJ cm −2 , time delay: 1.3 ps). Full size image The sample was pumped with an infrared (IR) pulse at 800 nm wavelength and with 70 fs (FWHM) pulse duration. The wavelength of the soft X-ray probe pulse was tuned to 20.8 nm corresponding to the Co 3 p 3/2 absorption resonance, which exhibits magnetic scattering contrast due to the X-ray magnetic circular dichroism effect [13] , [14] , [15] . Sensitivity to the spatial response during the demagnetization was obtained via the observation of small-angle X-ray scattering (SAXS) of the probe pulse. The SAXS pattern was detected on a 2D detector and investigated as a function of the pump-probe delay and pump-laser fluence, as sketched in Fig. 1 and described in the Methods. For SAXS from magnetic domain patterns with X-ray magnetic circular dichroism contrast, the scattered intensity is known to be proportional to the square of the local sample magnetization vector M projected onto the propagation vector k of the incident circularly polarized X-rays. Linearly polarized light, as used in our experiment, can be perceived as a superposition of left- and right-circularly polarized X-rays that have identical scattering cross-sections [14] . The magnetic SAXS cross-section is composed of the structure factor reflecting the periodicity of the domain arrangement and of the magnetic form factor describing the mean magnetization profile of the domains, especially at the domain walls [14] , [16] (see Supplementary Discussion ). As evidenced by the azimuthal symmetry of the SAXS ring for our magnetic system, the ensemble-average properties of the magnetic domain pattern are laterally isotropic, and we evaluate the radial scattering distribution as a function of the magnitude of the momentum transfer q after integration over the azimuthal angle Φ ( Fig. 1b ). By fitting the intensity distribution, we determine the maximum intensity and hence the corresponding momentum transfer value for the modal value q peak of the distribution. The square root of the maximum scattering intensity serves as a measure of the average domain magnetization magnitude M (ref. 14 ). Ultrafast demagnetization and spatial response In Fig. 2a , we present the normalized magnetization magnitude as a function of IR pump fluence and pump-probe delay. These results reproduce observations made previously for the demagnetization of single-domain Ni (refs 1 , 4 ), Co (ref. 4 ), and in particular CoPd (ref. 3 ), thin films obtained by other experimental approaches: an ultrafast drop of the magnetization is observed with a time constant in the femtosecond regime, followed by a slow recovery of the magnetization on the picosecond timescale. The temporal resolution of 240 fs (FWHM) in our experiments is dominated by the arrival time jitter between the optical and the soft X-ray pulse. Lines represent a phenomenological fit to the experimental data consisting of three different exponential decays convolved with the temporal resolution, relating to the ultrafast demagnetization, fast recovery and long-time recovery from the quenched state [3] . For the initial ultrafast demagnetization, we achieve good fit results for a demagnetization time constant ≤300 fs for all pump fluences. Subsequently, we observe a relatively fast but partial recovery of the magnetization within the first 2 ps with time constants in the range from (0.6±0.2) ps (IR pump with 7.9 mJ cm −2 fluence) to (1.3±0.4) ps (14.2 mJ cm −2 ) followed by a slow recovery process with tens of picoseconds time constants. 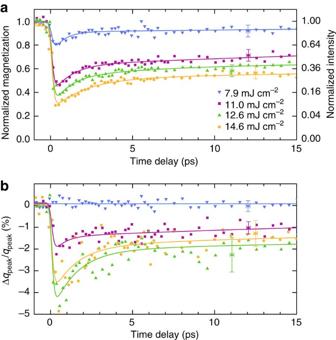Figure 2: Ultrafast response of the magnetic system to the femtosecond IR pump. (a) Evolution of the intensity and (b) shift of the SAXS distribution's modal value in dependence on the pump-probe delay. The square root of the intensity serves as a measure for the domain's magnetization. Each data point is normalized to a SAXS measurement taken without pump. The typical error is indicated at a single data point for each time course. The time delay error is given by the time resolution of the experiment. The error of the normalized intensity and the peak shift were taken from the fit of the SAXS profile. The lines are fits to the data using the sum of three exponentials convolved with the time resolution of the experiment. Figure 2: Ultrafast response of the magnetic system to the femtosecond IR pump. ( a ) Evolution of the intensity and ( b ) shift of the SAXS distribution's modal value in dependence on the pump-probe delay. The square root of the intensity serves as a measure for the domain's magnetization. Each data point is normalized to a SAXS measurement taken without pump. The typical error is indicated at a single data point for each time course. The time delay error is given by the time resolution of the experiment. The error of the normalized intensity and the peak shift were taken from the fit of the SAXS profile. The lines are fits to the data using the sum of three exponentials convolved with the time resolution of the experiment. Full size image Our main experimental result is shown in Fig. 2b . Here, we present the relative change Δ q peak / q peak of the SAXS distribution's modal value as a function of pump fluence and pump-probe delay. We observe a decrease of q peak of the pumped system relative to the unpumped system on the femtosecond timescale, indicating an ultrafast spatial response of the domain system on sub-100 nm lengthscales, which is observed for the first time. The temporal behaviour is similar to that of the magnetization change, and we therefore fitted the spatial-response delay-time course analogously to the demagnetization. We observe an ultrafast decrease of q peak with time constants below 300 fs towards a minimum located at about 0.5 ps, followed by a fast but only partial recovery of q peak . The recovery time constants are, within the experimental error, equal to the time constants observed for M . For the largest pump fluences around 14 mJ cm −2 , we observe a maximum shift of Δ q peak / q peak =(4±1)% to smaller q values, whereas we cannot detect any change for the lowest pump fluence of 7.9 mJ cm −2 . Given the inverse relationship ξ =2 π / q between the magnetic in-plane correlation length ξ in real space and the momentum transfer q in reciprocal space, such a contraction of the SAXS pattern as evidenced via Δ q peak / q peak by 4% would correspond to an expansion of the in-plane correlation length by the same ratio. In this picture, the average width of all up and down domains would increase by 2.8 nm during 0.5 ps within the entire probed area of (250×250) μm 2 . If homogeneous throughout the sample, such a hypothetical process must involve a rearrangement of domain boundaries over distances corresponding to 4% of the linear field of view, that is, 10 μm within 0.5 ps. This would correspond to domain wall velocities on the order of 10 7 m s −1 . If a domain growth process would occur in a hypothetic, inhomogeneous fashion such that selected domains were entirely annihilated or the domain width distribution was significantly broadened, a domain wall motion over a few nanometres would have to occur in the sub-picosecond regime, necessitating domain wall speeds on the order of 10 4 –10 5 m s −1 . This speed is orders of magnitude higher than reported domain wall motion in magnetic fields [17] or due to spin currents [18] and exceeds the group velocity and even the phase velocity of magnons [19] . We can thus rule out explanations of the observed effect based on domain wall motion driven by Landau–Lifshitz–Gilbert dynamics simply due to the fact that the resulting lateral propagation speed is too slow. On the same ground, a thermal expansion effect can be excluded, given speeds of sound below 10 4 m s −1 for both Co and Pt. Hence, the key question is which mechanism can explain the observed ultrafast spatial response. We propose that spin-dependent transport of the optically excited electrons across the domain walls in our purely ferromagnetic system can provide such a mechanism. Experimental evidence of interlayer spin transfer has recently been reported for a FM–PM–FM system with ferromagnetic versus antiferromagnetic interlayer exchange coupling [6] . The concept of superdiffusive spin transport has recently been invoked in a theoretical study of optically pumped electrons at the FM–PM interface, with velocities of electrons optically excited into the sp -bands on the order of 10 6 m s −1 (ref. 7 ). It is based on the notion that the lifetimes, velocities and, consequentially, the mean free paths for hot electrons in metals are spin dependent if the electrons move in a magnetized region and that secondary electrons generated in scattering events can contribute significantly to the resulting spin currents. Recent work on ballistic versus diffusive transport of spin-polarized electrons through thin epitaxial gold films is in line with this concept [20] . As the mean free path of low-energy excited electrons in metals is on the order of a few nanometres, the spin-dependent electron transport does not only play a role for interlayer spin exchange between thin metal films but also has to be taken into account for magnetic systems that are laterally structured on the nanometre scale. To corroborate if superdiffusive spin transport can be responsible for our experimental observations, we performed simulations of the lateral spin diffusion based on the work of Battiato et al . [7] . We applied a Monte–Carlo simulation approach to account for the irregular lateral domain pattern of our sample. As a representative magnetization map, we used a binarized magnetic force microscopy image of our sample similar to the one presented in Fig. 1a , neglecting the width of the domain walls. As a further simplification, the simulation was performed on a two-dimensional lattice and spin-diffusion components in the direction of the sample normal were ignored (for simulation details, see Methods ). Analogous to the results of the FM–PM simulation in ref. 7 , we observe a strong accumulation of minority electrons at the FM–FM domain boundaries. For our case of a system in which the topology is purely defined by magnetic order via domain walls separating oppositely magnetized domains, this results in a softening of the magnetization profile at the domain walls ( Fig. 3a,b ). By Fourier-transforming the magnetization maps obtained in the simulation for different times after the initial optical excitation, we simulate the pump-probe SAXS experiment. The model reproduces the drop in the scattering intensity and shift in the q peak position ( Fig. 3c ). As sketched in Fig. 3d , this shift is directly related to a dramatic change of the domain's scattering form factor induced by the smoothing of magnetization profile at the domain walls. When the magnetization profile at the domain walls significantly softens, the corresponding scattering form factor decreases much faster with increasing scattering vector compared with the scattering factor of a thin and steep domain wall (for an explanation of the magnetic scattering factor, see the Supplementary Discussion ). As a result, the structure function peak, which is strongly broadened reflecting the distribution of correlation lengths in the domain arrangement, will be deformed during spin diffusion in the domain system and the position of the scattering intensity maximum shifts. As this process is highly non-linear, a significant shift is observed only for high pump fluences. In our simulation model, we observe a broadening of the domain interface on the order of 20 nm (FWHM). 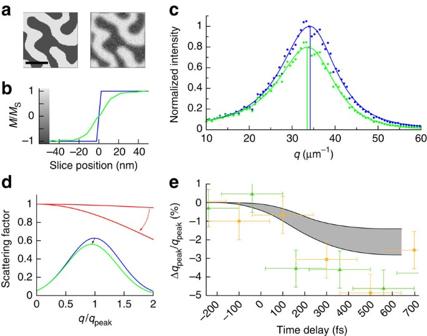Figure 3: Results from Monte–Carlo simulation of superdiffusive spin-transport. (a) Temporal evolution of the magnetization in a selected real-space region (scale bar, 200 nm) at the start of the simulation (left panel) and after 300 fs (right panel). (b) Magnetization profiles at a domain boundary extracted from the magnetization maps. The blue line corresponds to the initial condition, the green line shows the situation after 300 fs. (c) Simulated azimuthally integrated SAXS spectrum generated from the initial magnetization map (blue points) and after 300 fs (green points). Fits (lines) were performed analogously to the ones of the experimental data. (d) Schematic explanation of the observed peak shift. Because of the softening of the magnetization profile at the domain walls during spin diffusion, the corresponding scattering form factor (red line) decreases much faster with increasing scattering vector compared with the initial scattering factor of a thin and steep domain wall. As a result, the broadened first-order magnetic structure peak in equilibrium (blue line) will be deformed after the pump (green line) and the position of the intensity maximum shifts. (e) Temporal evolution of the SAXS peak shift in the simulation (lines) and in the experiment (points and error bars taken fromFig. 2). The shaded area symbolizes the estimated confidence interval of the numeric results, considering the uncertainties in the input parameters to the simulation. Because of a convolution of the simulation data with the experimental time resolution, a shift is already present before time zero. Figure 3: Results from Monte–Carlo simulation of superdiffusive spin-transport. ( a ) Temporal evolution of the magnetization in a selected real-space region (scale bar, 200 nm) at the start of the simulation (left panel) and after 300 fs (right panel). ( b ) Magnetization profiles at a domain boundary extracted from the magnetization maps. The blue line corresponds to the initial condition, the green line shows the situation after 300 fs. ( c ) Simulated azimuthally integrated SAXS spectrum generated from the initial magnetization map (blue points) and after 300 fs (green points). Fits (lines) were performed analogously to the ones of the experimental data. ( d ) Schematic explanation of the observed peak shift. Because of the softening of the magnetization profile at the domain walls during spin diffusion, the corresponding scattering form factor (red line) decreases much faster with increasing scattering vector compared with the initial scattering factor of a thin and steep domain wall. As a result, the broadened first-order magnetic structure peak in equilibrium (blue line) will be deformed after the pump (green line) and the position of the intensity maximum shifts. ( e ) Temporal evolution of the SAXS peak shift in the simulation (lines) and in the experiment (points and error bars taken from Fig. 2 ). The shaded area symbolizes the estimated confidence interval of the numeric results, considering the uncertainties in the input parameters to the simulation. Because of a convolution of the simulation data with the experimental time resolution, a shift is already present before time zero. Full size image In Fig. 3e , we compare the time evolution of the q peak position shift in the simulation with our experimental data as presented in Fig. 2 . Our model explains the sign, the timescale and—taking into account the large experimental error bars and the strong simplifications of the model—the magnitude of the experimentally observed shift of the SAXS distribution's modal value. Note that in contrast to the geometry in ref. 6 , no interfaces between chemically different materials are present, and in contrast to ref. 7 , it is the spin diffusion within the 2D sample plane producing the demagnetizing effect. In particular, no gradient in the hot-electron density due to the variation of the locally absorbed IR power with penetration depth, as always present in vertically layered systems, is required for this mechanism. Furthermore, the spin separation at the domain boundaries is, in particular, caused by the spin-dependent diffusion properties and cannot be explained by a simple intermixture of hot carriers at the domain walls, as the excitation rate in the simulation is independent of the electron spin. We have considered the ultrafast change in magnetic anisotropy recently reported by Boeglin et al . [3] as an alternative mechanism inducing a change of the domain wall magnetization profile. The authors in ref. 3 find a 29% change of orbital moment, which can be correlated with an anisotropy change [21] . Making conservative assumptions, we have carried out micromagnetic simulations with a 50% reduced anisotropy at t =0, taking the dynamic change in saturation magnetization as evident in Fig. 2 into account. Using a Landau–Lifshitz–Gilbert time evolution, the resulting magnetization profile changes by 1.2 nm after a duration of 1 ps (see Methods and Supplementary Fig. S2 ). The resulting effect is clearly too small to explain the observations in our experiment. While our simulation clearly shows the origin of the spatial response, the total amount of demagnetization is underestimated as the simulation neglects spin diffusion perpendicular to the sample plane [7] and excludes additional spin-flip channels, for example via electron–phonon scattering [4] . More sophisticated theoretical modelling including the multilayer structure of the thin magnetic film and the widths of domain walls, details of the electronic band structure and in particular spin-dependent inelastic electron scattering will have to be developed in the future and can be expected to lead to a better understanding of the effects of electronic magnetization transport in magnetic nanostructures. The observation of a spatial response of a ferromagnet—connected to the presence of domain walls—in response to femtosecond optical pulses lends support to the predicted importance of superdiffusive spin transport in magnetically heterogeneous systems and illustrates the generality of this concept beyond FM–PM interfaces [6] , [7] . We note that the spatio-temporal scale of the observed effects is in line with the recent observation of ballistic and diffusive spin transport channels [20] , when taking into account the non-epitaxial nature of our samples. As nanoscale heterogeneity is an intrinsic feature of many material systems, ultrafast effects based on preferential electron transport at inhomogeneities may be of general importance. Given the tremendous advances in the use of magnetic interfaces for electronic and spintronic applications in the past decades, one may envision the utilization of superdiffusive spin transport across ferromagnetic domain walls for ultrafast magneto-optical devices in the future. We anticipate that it will be possible to tailor time constants of optical demagnetization by variation of the domain size when approaching the spin-diffusion lengthscale. Sample fabrication The Co/Pt multilayers with a composition of Pt(50)/[Co(8)/Pt(14)] 16 /Pt(6) (Å) were deposited on 50-nm-thick Si 3 N 4 membranes via ion-assisted DC magnetron sputtering [22] . By out-of-plane demagnetization before the experiment, the system is conditioned into a remanent labyrinth-domain state, which was characterized via SAXS at the BESSY II synchrotron source as well as by magnetic force microscopy. Pump-probe experiments Experiments were carried out at beamline BL3 of the FEL facility FLASH in Hamburg, Germany. The X-ray probe pulse (20.84 nm) with a natural spectral bandwidth of about 1% was only moderately focused down to a spot size of 650 μm (FWHM) on the sample. We estimate an energy density of (2.0±0.6) mJ cm −2 at the sample, which is below the damage threshold determined earlier [15] . The IR (800 nm) pump pulse was delivered by a Ti:sapphire based laser system, which is electronically synchronized to the FEL accelerator [23] . A small parallax between X-ray and IR beam of 3° results in a temporal broadening of 43 fs. The focus of the pump laser was set to 1.20×0.94 mm 2 (FWHM) ensuring nearly homogeneous pumping of the whole X-ray transparent sample area of 250×250 μm 2 . The duration of the pump pulse was 70 fs (FWHM) and about 100 fs for the probe pulse. The arrival time jitter distribution between the IR and the X-ray pulses had a width of approximately 200 fs (FWHM) resulting in a total calculated time resolution of the experiment of 240 fs. The magnetic SAXS experiments were performed in transmission geometry ( Fig. 1a ) with a charge-coupled device (CCD) area detector (2,048×2,048 pixels, 13.5×13.5 μm 2 pixel size) placed 55 mm behind the sample. The maximum detected scattering angle corresponds to ~60 nm real-space distances, but changes in the ensemble-average properties of the magnetic topography can be detected with 3 nm accuracy as described below. The intense directly transmitted radiation was blocked by a central beamstop. The CCD was IR protected by a 250-nm-thick Al filter. Taking the filter transmission and the quantum efficiency of the detector into account, the system had an X-ray detection efficiency of 30%. For each pump-probe time delay, two SAXS patterns, first without and then with pump pulse, were recorded from three integrated single-shot pump-probe intervals at 1 Hz repetition rate. The pump energy density on the sample was varied between (7.9±1.1) mJ cm −2 and (14.2±2.0) mJ cm −2 . SAXS data treatment The SAXS spectra as shown in Fig. 1b were retrieved by azimuthal integration of the 2D patterns after background subtraction and masking of beamstop shadow and charge scattering streaks from the membrane edges. All intensities were normalized to the charge-scattering signal from the membrane edges. Additional charge scattering was removed from the spectra by fitting a q −4 dependency to the intensity data at very low q where the magnetic signal is small compared with the charge scattering. The residual magnetic spectra were fitted with a split Pearson type VII distribution, which is a class of distributions that accounts for the skewness and kurtosis of natural distributions. In our case, the analytical fit function reads: with different parameter sets ( α 1 , m 1 ) and ( α 2 , m 2 ) for the left and the right side of the mode q peak . The procedure results in 3 nm spatial resolution in the detection of changes of the in-plane correlation length. The delay-scan graphs in Fig. 2 were drawn from the peak intensity ( I 0 ) values obtained from the measurements with IR pump ( I pumped ( t )) at a time delay Δ t = t − t 0 normalized to the unpumped spectra ( I unpumped ). The delay scans were fitted with the sum of three different exponentials convolved with the time resolution ( σ t ) of the experiment (Gaussian distribution): A demag , A recov1 and A recov2 denote the strength of the demagnetization and the recovery process, respectively, whereas τ demag , τ recov1 and τ recov2 denote the time constants of these processes. H ( t ) is the Heaviside step function ( H ( t )=1 if t >0, H ( t )=0 elsewhere). The time zero ( t 0 ) was obtained from the fit. The change in the intensity peak position ( q peak ) is calculated analogously as Δ q peak / q peak =( q pumped − q unpumped )/ q unpumped and is fitted with three exponentials as described for the intensity change. Monte-Carlo simulation The simulation starts at time zero with a number of 0.1 excited electrons per atom corresponding to a pump fluence of approximately 14 mJ cm −2 with an equal fraction of spin-up and spin-down electrons independent of the local sample magnetization. The energy of the hot electrons is equally distributed over those previously unoccupied electronic states between the Fermi energy and the highest optically accessible state (1.55 eV above the Fermi edge). For each simulation run, the electron cascades initiated from 1.7×10 7 primarily excited electrons were simulated in a lateral sample plane with a physical size of 10×10 μm 2 . The magnetization maps had a spatial resolution of 4.88×4.88 nm 2 . The spin- and energy-dependent inelastic electron lifetimes were taken from experimental data for Cobalt [24] , [25] , the Co electron velocities and all parameters for Pt from ab initio calculations [26] , [27] . The lifetimes ( τ inel ) and velocities are discretized in channels of 0.1 eV width and averaged according to the composition of the multilayer. During the subsequent temporal evolution, we assume no interaction between the hot electrons and feedback of the hot electron gas on the parameters of the simulation is neglected as well. Without such self-consistent feedback, we expect our simulation to be valid only for the first hundreds of femtoseconds of the demagnetization process. After time zero, the electrons move in isotropically distributed directions on a straight-line trajectory up to an elastic or inelastic scattering event. The positions are updated in time steps of t MC =1 fs. In case of inelastic scattering events, secondary electrons are generated with isotropically distributed, random momentum direction. The spin of the secondary electrons is chosen randomly independent of the scattered electron and of the local magnetization. The energy of the scattered electrons is calculated from classical two-particle collision [7] , [28] . The elastic scattering probability (Ω el ) is calculated from the inelastic probability (Ω inel = t MC / τ inel ) as Ω el = a Ω inel with the constant a ranging from 0.5 to 2 for different MCS runs. Additional inelastic contributions, for example from phonon scattering are neglected. As a result of the electron-electron scattering, the electron gas thermalizes. Every 50 fs, a magnetization map considering the position of the migrating electrons is saved assuming an initial magnetization of 1 μ B per atom [29] . The motion of the electrons is strongly affected by the local magnetization. As detailed by Battiato et al . [7] , majority electrons possess a larger mean-free path length compared with minority electrons. If, however, a majority electron crosses a domain boundary, it will become a minority electron within the new domain and it is therefore trapped in the vicinity of the domain wall. As a result, these cascades of spin-polarized electrons within a landscape of ferromagnetic domains cause an enhanced demagnetization at the domain boundaries due to an accumulation of minority electrons. Micromagnetic simulations Micromagnetic simulations of the impact of a change in the magnetocrystalline anisotropy were carried out using the OOMMF software [30] , based on dynamics using the Landau–Lifshitz–Gilbert (LLG) equation. A 3D 300×300×36 nm 3 simulation of a domain pattern was carried out with a cell size of 1×1×4 nm 3 and the resulting magnetization profile between adjacent domains was extracted. Values for the uniaxial anisotropy and the saturation magnetization have been taken from ref. 29 . In the simulation, an equilibrium domain-wall width of 6.2 nm is yielded. Starting from the equilibrium domain configuration at t =0, the anisotropy is reduced by 50% and the saturation magnetization by 70%. After 1 ps of LLG evolution, the domain wall broadens by 1.2 nm ( Supplementary Fig. S2 ). How to cite this article: Pfau, B. et al . Ultrafast optical demagnetization manipulates nanoscale spin structure in domain walls. Nat. Commun. 3:1100 doi: 10.1038/ncomms2108 (2012).